Removal of stacking-fault tetrahedra by twin boundaries in nanotwinned metals Stacking-fault tetrahedra are detrimental defects in neutron- or proton-irradiated structural metals with face-centered cubic structures. Their removal is very challenging and typically requires annealing at very high temperatures, incorporation of interstitials or interaction with mobile dislocations. Here we present an alternative solution to remove stacking-fault tetrahedra discovered during room temperature, in situ Kr ion irradiation of epitaxial nanotwinned Ag with an average twin spacing of ~8 nm. A large number of stacking-fault tetrahedra were removed during their interactions with abundant coherent twin boundaries. Consequently the density of stacking-fault tetrahedra in irradiated nanotwinned Ag was much lower than that in its bulk counterpart. Two fundamental interaction mechanisms were identified, and compared with predictions by molecular dynamics simulations. In situ studies also revealed a new phenomenon: radiation-induced frequent migration of coherent and incoherent twin boundaries. Potential migration mechanisms are discussed. Neutron, proton or heavy ion irradiation can create a large amount of defect clusters, including bubbles, voids and dislocation loops in irradiated metallic materials. Consequently, radiation may lead to void swelling and degrade the mechanical properties of metallic materials in terms of radiation hardening, embrittlement and irradiation-induced creep. Various types of defect sinks, such as grain boundaries and interphase interfaces, have been used to reduce the density of radiation-induced defects [1] , [2] , [3] , [4] . King and Smith [5] studied the mechanism of point defect absorption by grain boundaries and ∑3 {111} coherent twin boundaries (CTBs) in electron-irradiated Al and Cu, and showed that twin boundaries may be biased sinks for dislocation loops. Recently, there are increasing interests on radiation tolerance of nanostructured materials because they possess a significant fraction of high-angle grain boundaries that lead to reduction of radiation-induced defect density [6] , [7] . Atomistic modelling has also been adopted to investigate the radiation response of high-angle grain boundaries in nanomaterials [8] , [9] , [10] . Molecular dynamics (MD) simulations of Σ11 grain boundaries in face-centered cubic (fcc) Cu showed that radiation-induced interstitials were first absorbed by grain boundaries to form interstitial-rich (or interstitial-loaded) grain boundaries that promote the vacancy-interstitial recombination. Compared with pristine grain boundaries, the interstitial-rich grain boundaries reduce the barrier for interstitial emission and thus emitted interstitials (from grain boundaries) can effectively annihilate vacancies in the grain interior [11] . Meanwhile the interstitial-rich grain boundaries also reduce the vacancy diffusion barrier so that it is easier for vacancies to migrate to grain boundaries where they recombine with interstitials. Besides high-angle grain boundaries, layer interfaces in certain immiscible metallic multilayers [12] , [13] , [14] , [15] also act as remarkable sinks for point defects, and lead to dramatic reduction of defect density, swelling and radiation hardening. MD simulations showed that Cu/Nb layer interfaces can act as inexhaustible sinks for radiation-induced point defects [16] . Stacking-fault tetrahedra (SFTs) are a dominant type of vacancy cluster in various irradiated fcc metals with low-to-intermediate stacking fault energy (SFE) [4] , [17] , [18] in the absence of noble gases in the materials. SFTs, once formed via collapse of vacancy clusters [19] , [20] , are typically very stable, and their removal requires annealing at very high temperature [21] , incorporation of interstitials via radiation [19] or mobile dislocations [22] . Effective removal of high-density SFTs is necessary to minimize void swelling and alleviate radiation hardening. Recently, Niewczas and Hoagland [23] simulated the interaction between ∑3 {111} CTBs and SFTs, and found that the interaction led to destabilization of parent SFTs and production of new defects at twin boundaries. But their prediction received little attention as the proposed interactions require frequent migration of Shockley partials and twin boundaries, which occurs only sporadically in conventional bulk metallic materials with coarse grains. Hence, there is no experimental evidence to verify their predicted SFT removal mechanism to date. Meanwhile nanotwins have been shown to induce remarkably high mechanical strength in Cu, Ag and 330 stainless steel [24] , [25] , [26] , [27] , and twin boundaries are mobile under stress or annealing [28] , [29] . But little is known experimentally on radiation response of nanotwinned (nt) materials [30] . Here, we report on an in situ study of radiation damage in epitaxial nt Ag films in a transmission electron microscope at room temperature. Significant findings include twin thickness-dependent reduction of dislocation loop density, destruction of SFTs by twin boundaries and consequently drastic reduction of density of SFTs. Besides the validation of two SFT removal mechanisms predicted by MD simulations, we observed radiation-induced migration of coherent and incoherent twin boundaries (ITBs). These findings provide important implications for the design of swelling-resistant structural materials, and offer basis for exploration of physics of radiation-induced twin boundary migrations. Microscopic overview of irradiated nt Ag films As-deposited Ag films have high-density growth twins ( Supplementary Fig. S1a–b ) with Σ3{111} CTBs and Σ3{112} ITBs with an average twin spacing ( t ave ) of 8 and 70 nm, respectively. The average thickness of twins is identical to that of matrix, that is twins account for 50 vol.% of the films. The as-deposited nt Ag had a low defect density in the range of 10 19 –10 20 m −3 ( Supplementary Fig. S1c–d ). These defects were dislocation loops and threading dislocations that were generated during deposition or specimen preparation. We did not observe any SFTs from bright-field or weak-beam dark-field cross-sectional transmission electron microscopy (XTEM) experiments. 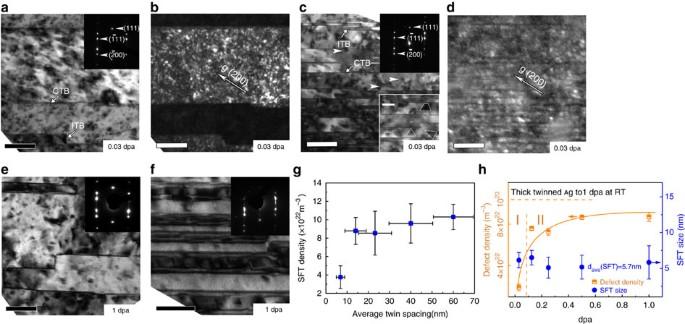Figure 1: Microscopy overview of defects and statistics of defect density in nanotwinned(nt) Ag films irradiated to different doses (a) Bright-field XTEM micrograph of thick twinned Ag with an average twin spacingtaveof 70 nm, irradiated to 0.03 displacement-per-atom (dpa) and examined along the Ag ‹011› zone axis, shows high density of ∑3 {111}CTBs and vertical ∑3{112}ITBs. High-density defects were generated by irradiation. Scale bar, 30 nm. (b) Corresponding dark-field image showing the formation of high-density defects. Scale bar, 30 nm. (c) Bright-field TEM micrograph of fine nt Ag (tave=8 nm) irradiated to 0.03 dpa shows significantly lower defect density than thick nt Ag. Irradiation led to triangular and trapezoidal stacking-fault tetrahedra (SFTs) (inset) and other defect clusters. Main scale bar, 30 nm; inset scale bar, 5 nm. (d) Corresponding dark-field image of nt Ag confirms that defect density is much lower than that of thick twinned Ag. Scale bar, 30 nm. At 1 dpa, the density of defects in thick nt Ag (e) continued to increase and was much greater than fine nt Ag (f). The inserted selected area diffraction (SAD) pattern in (f) shows much stronger intensity of streaking lines, implying the formation of a high density of stacking faults, which were observed along twin boundaries. Scale bars, 30 nm. (g) The density of SFTs decreased sharply at smaller average twin spacing (8 nm).All specimens were irradiated up to 1 dpa. (h) Density of defects (including SFTs and dislocation loops) in thick twinned Ag increased sharply and reached saturation at 0.01 dpa (as shown by the horizontal dash line). In comparison, the density of defects in fine nt Ag (tave=8 nm) increased gradually by ~0.1 dpa in stage I, and then leveled off thereafter in stage II (0.1–1 dpa) to a lower saturation value, at least 50% lower than that of thick twinned Ag. The average size of SFTs remained constant, ~5.7 nm, throughout the irradiation experiment. The error bars represent s.d.’s. Figure 1a shows a bright-field XTEM micrograph of nt Ag films with t ave of 70 nm, irradiated by Kr ions up to a dose of 0.03 displacements-per-atom (dpa). High-density nanotwins with sharp twin boundaries were observed throughout the specimen. The inserted selected area diffraction pattern in Fig. 1a also provides clear evidence for the existence of Σ3{111} lateral CTBs. High-density dark spots, which are signatures of radiation-induced defect clusters, were also observed in the corresponding dark-field TEM image in Fig. 1b . In comparison, nt Ag with t ave of ~8 nm irradiated at the same condition had a much lower density of defect clusters as shown in Fig. 1c . Numerous SFTs were produced by radiation as indicated in the inset of Fig. 1c . The bases of SFTs were parallel to the CTBs and some SFTs were apparently truncated. Extra diffraction spots in selected area diffraction pattern arose from Σ3{112} ITBs as observed previously in as-deposited nt Ag and Cu [26] , [31] . Radiation at 0.25 dpa led to significant increase in defect density in the thick nt Ag, whereas the defect density in the fine nt Ag only increased moderately ( Supplementary Fig. S2 ). Figure 1: Microscopy overview of defects and statistics of defect density in nanotwinned(nt) Ag films irradiated to different doses ( a ) Bright-field XTEM micrograph of thick twinned Ag with an average twin spacing t ave of 70 nm, irradiated to 0.03 displacement-per-atom (dpa) and examined along the Ag ‹011› zone axis, shows high density of ∑3 {111}CTBs and vertical ∑3{112}ITBs. High-density defects were generated by irradiation. Scale bar, 30 nm. ( b ) Corresponding dark-field image showing the formation of high-density defects. Scale bar, 30 nm. ( c ) Bright-field TEM micrograph of fine nt Ag ( t ave =8 nm) irradiated to 0.03 dpa shows significantly lower defect density than thick nt Ag. Irradiation led to triangular and trapezoidal stacking-fault tetrahedra (SFTs) (inset) and other defect clusters. Main scale bar, 30 nm; inset scale bar, 5 nm. ( d ) Corresponding dark-field image of nt Ag confirms that defect density is much lower than that of thick twinned Ag. Scale bar, 30 nm. At 1 dpa, the density of defects in thick nt Ag ( e ) continued to increase and was much greater than fine nt Ag ( f ). The inserted selected area diffraction (SAD) pattern in ( f ) shows much stronger intensity of streaking lines, implying the formation of a high density of stacking faults, which were observed along twin boundaries. Scale bars, 30 nm. ( g ) The density of SFTs decreased sharply at smaller average twin spacing (8 nm).All specimens were irradiated up to 1 dpa. ( h ) Density of defects (including SFTs and dislocation loops) in thick twinned Ag increased sharply and reached saturation at 0.01 dpa (as shown by the horizontal dash line). In comparison, the density of defects in fine nt Ag ( t ave =8 nm) increased gradually by ~0.1 dpa in stage I, and then leveled off thereafter in stage II (0.1–1 dpa) to a lower saturation value, at least 50% lower than that of thick twinned Ag. The average size of SFTs remained constant, ~5.7 nm, throughout the irradiation experiment. The error bars represent s.d.’s. Full size image Morphology and density evolution of SFTs Detailed microstructural examination of nt Ag irradiated to 1 dpa also revealed several important characteristics. First, smaller twin spacing led to fewer SFTs. Fewer defects, and in particular fewer SFTs, were formed in the fine nt Ag ( Fig. 1f ) than that in the thick nt Ag ( Fig. 1e ). Besides bright-field TEM, extensive dark-field TEM and high resolution TEM (HRTEM) studies were also performed to identify SFTs and determine their density ( Supplementary Fig. S3 ). Second, many truncated SFTs were observed. Third, stacking faults (SFs) were observed frequently next to twin boundaries and inside twins in both fine and thick twinned Ag, and the existence of SFs was also confirmed by both elongated diffraction dots and streaking lines in the insets of Fig. 1e . Under the current imaging condition, it is SFs rather than SFTs that lead to the formation of streaking lines in the diffraction pattern. Statistics in Fig. 1g shows the density of SFTs reduced gradually with decreasing twin spacing down to ~15 nm, and was significantly lower when t <10 nm. Furthermore in Kr ion-irradiated nt Ag ( t ave =8 nm), the density of defects (including SFTs and dislocation loops) increased with dose rapidly before 0.1 dpa ( Fig. 1h ) and saturated thereafter up to 1 dpa. Meanwhile, the thick nt Ag showed at least twice greater defect density ( Fig. 1h ), which saturated at a much lower dose (0.01 dpa) during in situ irradiation. The average dimension of SFTs remained 5–6 nm over 0.01–1 dpa ( Fig. 1h ). Comparison of fine nt Ag before and after radiation (1 dpa) shows that the t ave remains the same, ~8 nm (as shown in Supplementary Fig. S4 ). According to the Silcox and Hirsch model [32] , SFTs can evolve from Frank loops through the migration of Shockley partials and the formation of stair-rod dislocations. To understand the formation of SFTs, we first compare the energetics for the formation of perfect loops versus Frank loops in Ag. The size of SFTs is evaluated by their edge length ( L ). The loop radius ( r L ) is defined as the radius of the circum-circle of one tetrahedron face. The formation of a faulted loop is favoured over a perfect loop if the following criterion satisfies [19] where γ SFE is the SFE, which is ~17 mJ m −2 for Ag [33] , μ is the shear modulus, b is the Burgers vector, ν is the Poisson’s ratio and r c is the dislocation core radius. For Ag, μ =30 GPa, b =0.289 nm, ν =0.37, r L =3.3 nm (calculated with L =5.7 nm, as shown in Fig. 1h ) and r c =1 nm, the right side of the equation thus becomes 25 mJ m −2 , greater than 17 mJ m −2 . Therefore the formation of Frank loop is energetically favourable over a perfect loop in Ag and consequently a considerable amount of SFTs were formed in irradiated Ag films. Furthermore, it was found that SFTs in various irradiated fcc metals (Ag, Au, Cu and Ni) are predominantly vacancy clusters [34] , [35] . The evolution of defect density with dose can be divided into two stages: rapid increase in stage I and saturation in stage II as shown in Fig. 1h . Stage I may arise from the formation of a large number of faulted loops during the initial stage of radiation. Defect density saturates in stage II because a balance between the rate of defect generation (by radiation) and removal (by twin boundaries) was established in nt Ag. Defect density in fine nt Ag ( t ave =8 nm) saturates at a level of 8 × 10 22 m −3 , as compared with 1.6 × 10 23 m −3 in Ag with thick twins ( t ave =70 nm) as shown by the dash line. Literature data on defect density of room temperature-irradiated Ag are scarce. Kiritani et al. [17] showed the density of SFTs in Ag irradiated by neutron at a similar dose at 573 K is ~1.5 × 10 22 m −3 , and reduction of radiation temperature by 100 K in Au (that has higher SFE and threshold displacement energy than Ag) can lead to an order of magnitude increase in defect density in Au. Also defect density in neutron-irradiated Ni and Cu at a similar dose level approaches 2–10 × 10 23 m −3 at room temperature [36] . Ag has a lower SFE than Au, Cu and Ni, and hence it is anticipated that the density of SFTs in bulk Ag irradiated at room temperature to a similar dose will be much greater than that observed in nt Ag. SFTs, the predominant type of vacancy clusters in irradiated Cu, Ni, Ag and Au [34] in the absence of noble gas, can expand (or shrink) by absorbing a vacancy (or an interstitial) or even collapse by consuming a sufficient number of interstitials [23] . Therefore, it is very important to note that a majority of SFTs in our study were actually annihilated through active interaction with twin boundaries as supported by several observations. First of all, direct evidence of annihilation of SFTs via their frequent interactions with twin boundaries was captured. Sequential video clips in Fig. 2 obtained from Supplementary Video S1 (from the area of red box highlighted in Supplementary Fig. S5 ) show that the apex of a 5 nm SFT touched a CTB, T a . The original SFT then split into two smaller SFTs after 2 s. The upper SFT, whose apex contacted the upper CTB, T b , disappeared by 5 s. Meanwhile the apex of the lower SFT was truncated by T a . The truncated SFT nearly disappeared by 10 s. Comparison shows the twin spacing (separation distance between T a and T b ) shrank from 8–7 nm, indicating that twin boundaries migrated during radiation from 0.075–0.081 dpa. Second, CTBs were severely distorted after interaction with SFTs as revealed by the formation of SFs along twin boundaries ( Fig. 1f ). Third, twin spacing has a significant influence on the density of SFTs, that is, the smaller the twin spacing, the lower the density of SFTs. Also, truncated SFTs were frequently observed adjacent to CTBs (the inset of Fig. 1c ). The annihilation mechanisms of SFTs by twin boundaries are briefly discussed as follows. 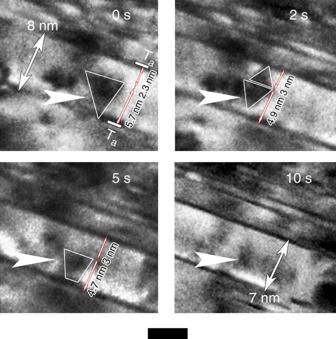Figure 2:In situobservation of SFTs interacting with CTBs over a dose range of 0.075–0.081 dpa. The apex of a 5 nm SFT was in contact with CTB Taat 0 s. The SFT split into two smaller SFTs joint from their bases at 2 s. By 5 s, the upper SFT adjacent to Tbvanished and the lower SFT was truncated from its tip. At 10 s, the SFT had a core barely discernible and the twin spacing shrank by 1 nm (seeSupplementary Video S1). (scale bar, 5 nm). Figure 2: In situ observation of SFTs interacting with CTBs over a dose range of 0.075–0.081 dpa. The apex of a 5 nm SFT was in contact with CTB T a at 0 s. The SFT split into two smaller SFTs joint from their bases at 2 s. By 5 s, the upper SFT adjacent to T b vanished and the lower SFT was truncated from its tip. At 10 s, the SFT had a core barely discernible and the twin spacing shrank by 1 nm (see Supplementary Video S1 ). (scale bar, 5 nm). Full size image The HRTEM image in Fig. 3a shows two truncated SFTs adjacent to CTBs. SFT-a was truncated from its apex and the destruction of SFT-b started from its base in contact with a lower CTB. Two possible annihilation mechanisms are illustrated in Fig. 3b . Atomistic simulations [23] , [37] have shown that when a mobile twin boundary reaches an SFT from its apex as depicted in the upper case in Fig. 3b , the SFT–twin boundary interaction transforms the {111} apex of SFT in matrix to a smaller {100} T tetrahedron residing temporarily within the twin lattice, which then collapses rapidly into a partial loop on the {111} plane in the twinned crystal. SFs also form next to the twin boundary. Continuous migration of the twin boundary towards the SFT leads to the further consumption of the truncated SFT. SFs absorb vacancies supplied by the SFT and continuously expand along the twin boundary. On the other hand, when the SFT is approached by a mobile twin boundary from its base as shown in the lower case of Fig. 3b , a mobile Shockley partial, a/6[121], migrating along the twin boundary could interact with stair-rod dislocations, AB (a/6[1 0]), AC (a/6[ 11]) and BC (a/6[ 01]), at the base of SFT. The interactions with AB and AC lead to new mobile Shockley partials (a/6[211] and a/6[112]) whose migration on ABD and ACD planes of the SFT can result in the unfaulting of Frank loops [18] . The two scenarios predicted by MD simulations are consistent with our in situ observations. Note that intensive SFT–twin boundary interactions result in high-density SFs, adjacent to twin boundaries as shown in Fig. 3c . Foregoing discussions strongly suggest that twin boundaries play a remarkable role during the removal of radiation-induced SFTs. 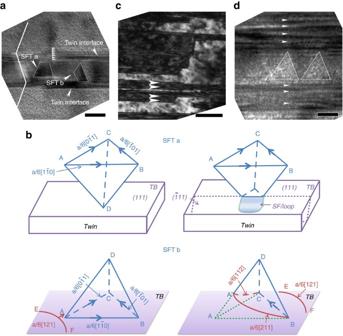Figure 3: High-resolution TEM of SFTs and their interaction mechanism with twin boundaries. (a) HRTEM image of two truncated SFTs during their interactions with CTBs. SFT-a was truncated from its apex, whereas SFT-b was destructed from its base. Scale bar, 4 nm. (b) Schematics of two types of interactions between SFTs and twin boundaries corresponding to the two cases in (a). The removal of SFT initiated from its apex (in contact with a twin boundary) results in the formation of dislocation loops on {111} plane in the twin lattices. In the lower case, the interaction of a mobile partial with stair-rod dislocations, AB and AC, results in two new mobile partials that can migrate on the surface of SFT and lead to its decomposition. (c) Stacking faults along twin boundaries in irradiated nt Ag (tave=8 nm) were induced by SFT–twin boundary interactions as shown by XTEM micrograph. Scale bar, 40 nm. (d) HRTEM micrograph showing the formation of groups of stacking faults in irradiated thin nt Ag (up to 1 dpa). Scale bar, 4 nm. Figure 3: High-resolution TEM of SFTs and their interaction mechanism with twin boundaries. ( a ) HRTEM image of two truncated SFTs during their interactions with CTBs. SFT-a was truncated from its apex, whereas SFT-b was destructed from its base. Scale bar, 4 nm. ( b ) Schematics of two types of interactions between SFTs and twin boundaries corresponding to the two cases in ( a ). The removal of SFT initiated from its apex (in contact with a twin boundary) results in the formation of dislocation loops on {111} plane in the twin lattices. In the lower case, the interaction of a mobile partial with stair-rod dislocations, AB and AC, results in two new mobile partials that can migrate on the surface of SFT and lead to its decomposition. ( c ) Stacking faults along twin boundaries in irradiated nt Ag ( t ave =8 nm) were induced by SFT–twin boundary interactions as shown by XTEM micrograph. Scale bar, 40 nm. ( d ) HRTEM micrograph showing the formation of groups of stacking faults in irradiated thin nt Ag (up to 1 dpa). Scale bar, 4 nm. Full size image What MD simulations did not capture though is that the continuous interactions led to the formation of multiple SFs along twin boundaries, and thus twin boundary appears ‘thicker’ after radiation. A thicker twin boundary increases the probability of its interaction with SFTs. In the fine nt Ag specimen ( Fig. 1f ), the volume fraction of irradiation-induced SFs is estimated to be ~10% using a method shown in Supplementary Fig. S6 . The kinetic interactions of SFTs with twin boundaries may also be enhanced by several other means. First, continuous growth of SFTs in size (before reaching a saturation dimension) coupled with smaller t ave may expedite their interactions. Second, twin boundaries may be mobile. In situ nanoindentation studies and MD simulations have shown that ITBs in nt Cu can migrate rapidly under stress or annealing through the movement of mobile Shockley partials [28] , [29] , [31] . The migration can lead to detwinning. However, there is no prior evidence on radiation-induced migration of twin boundaries. We have captured frequent migration of twin boundaries during in situ radiation studies (see Supplementary Video S2 ). TEM micrographs in Fig. 4 show an ITB in thick nt Ag ( t ave =70 nm) migrated by 5.7 nm during radiation from 0.5 to 1 dpa. Another example of such migration in irradiated fine nt Ag ( t ave =8 nm) is shown in Fig. 5 obtained from Supplementary Video S1 (focusing on the region highlighted by a yellow box in Supplementary Fig. S5 ). Area A consists of several ITBs as outlined and labelled as T1–T5. Snap shots were taken over the dose of ~0.07–0.11 dpa. As seen in the 0–15 s frames, the ITB T1 and T2 aligned well with each other. But T2 was completely removed by 25 s and a new ITB T3 forms and aligns with T1. By 35 s, T3 was separated from T4 (evolved from T1) and formed inclined ITBs. By 55 s, T3 migrated leftward by 2 nm and finally aligned with ITB T5. Two factors may lead to the formation and migration of new ITBs. First, the destruction of SFTs by CTBs leads to the formation of multiple SFs (as shown in Fig. 3c ). ITBs consist of groups of Shockley partials, one on each atomic plane [31] . The summation of Burgers vectors of three Shockley partials on three adjacent planes is zero [29] . Under stress, sharp ITBs can transform into diffuse boundaries (groups of wide SFs). It may be energetically favourable for the groups of SFs (formed by destruction of SFTs) to evolve into wide ITBs. Second, ITBs are sources for Shockley partials and sinks for point defects. Radiation-induced defect clusters, including SFTs, may attract or repel partials inside ITBs and lead to their migration. Significant mobility makes twin boundaries an attractive candidate for removing radiation-induced SFTs as well as other defects. The physical mechanisms and details of radiation-induced twin boundary migration require atomistic simulations. Although twin boundaries can actively remove SFTs in irradiated metallic materials, special precaution shall be applied as twin boundaries may become less effective in removing He-stabilized defects, such as He bubbles, as shown previously [30] . 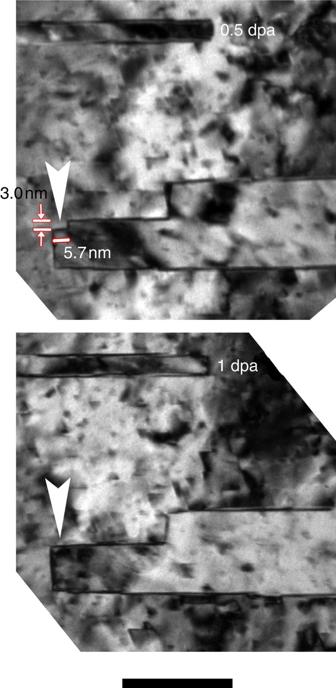Figure 4: Twin boundary migration in irradiated thick twinned Ag (tave=70 nm). Bright-field TEM micrograph shows a step consisted of an ITB (3 nm in height) and CTB (5.7 nm in width) segment as indicated by a white arrow. During continuous radiation (0.5–1 dpa), the ITB migrated left over a distance of 5.7 nm and consequently the step was removed (Supplementary Video S2). Scale bar, 40 nm. Figure 4: Twin boundary migration in irradiated thick twinned Ag ( t ave =70 nm). Bright-field TEM micrograph shows a step consisted of an ITB (3 nm in height) and CTB (5.7 nm in width) segment as indicated by a white arrow. During continuous radiation (0.5–1 dpa), the ITB migrated left over a distance of 5.7 nm and consequently the step was removed ( Supplementary Video S2 ). Scale bar, 40 nm. 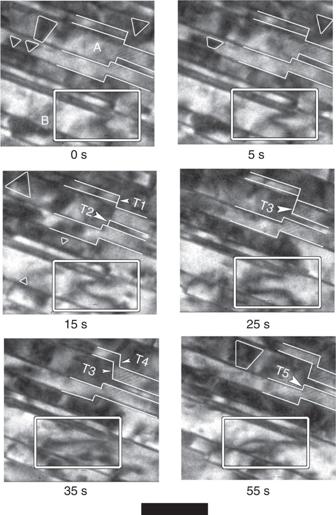Figure 5: Migration of twin boundaries in fine nt Ag (tave=8 nm). A series of TEM snapshots of irradiated Ag were captured over 0.07–0.11 dpa (Supplementary Video S1). Area A tracks the evolution of numerous ITBs (labelled as T), including the disappearance of T2 and migration of T3 and T4. By 55 s, T3 migrated leftward by ~2 nm. Area B (in the box) captures the emission of a dislocation (from an ITB) and its migration towards the opposite CTB. The migration of dislocation was confined by two twin boundaries. Scale bar, 20 nm. Full size image Figure 5: Migration of twin boundaries in fine nt Ag ( t ave =8 nm). A series of TEM snapshots of irradiated Ag were captured over 0.07–0.11 dpa ( Supplementary Video S1 ). Area A tracks the evolution of numerous ITBs (labelled as T), including the disappearance of T2 and migration of T3 and T4. By 55 s, T3 migrated leftward by ~2 nm. Area B (in the box) captures the emission of a dislocation (from an ITB) and its migration towards the opposite CTB. The migration of dislocation was confined by two twin boundaries. Scale bar, 20 nm. Full size image Other than twin boundaries, mobile dislocations may also interact with SFTs. The same in situ video ( Supplementary Video S1 ) also reveals the emission and migration of a dislocation as outlined in the box B in a series of snap shots in Fig. 5 . The dislocation in box B was emitted from an ITB at the beginning of the video during radiation and it evolved during continuous radiation. The migration of the dislocation was confined within the twins by attaching its upper end to the original ITB. The dislocation continued to propagate until it finally reached the lower CTB, where a dislocation loop formed by 55 s. Propagation of mobile dislocations may also contribute to the removal of some radiation-induced defects as shown previously [22] . Some of the well-known low-energy boundaries, such as CTBs, have long been considered ineffective defect sinks in irradiated metallic materials. However, this study suggests that CTBs and ITBs are critical to remove some of the most stable defect clusters (SFTs) induced by radiation. Thus, opportunities arise to design next-generation radiation-tolerant structural materials. Frequent migration of TBs is desirable to actively engage and remove SFTs, although mechanisms of radiation-induced TB migration requires further investigation via MD simulations. Epitaxial Ag films with thickness of ~2 μm were synthesized on Si (111) substrate by using DC magnetron sputtering technique at room temperature. XTEM specimens for in situ radiation study were prepared. Details of deposition and specimen preparation can be found elsewhere [26] . Before and post irradiation, the specimen was investigated by an FEI Tecnai G2 F20 ST microscope. The thickness of TEM foils was measured to be ~110 nm by using the Kossel–Mollenstedt fringes captured under two-beam conditions. Numerous specimens were irradiated with 1 MeV Kr ++ ions up to a maximum fluence of 2 × 10 14 ions m −2 (corresponding to a maximum of 1 dpa) at room temperature at the IVEM-TANDEM facility at Argonne National Laboratory where an ion accelerator is attached to a HITACHI H-9000NAR microscope. Depth-dependent damage and defect concentration profiles were calculated by the Stopping and Range of Ions in Matter (SRIM)-2008 [38] using a threshold energy of 40 eV for Ag. The density of defects, defined as the number of defects per unit volume, was estimated from abundant bright-field and dark-field TEM images. How to cite this article: Yu, K. Y. et al. Removal of stacking-fault tetrahedra by twin boundaries in nanotwinned metals. Nat. Commun. 4:1377 doi: 10.1038/ncomms2382 (2013).